Pathogen effector recognition-dependent association of NRG1 with EDS1 and SAG101 in TNL receptor immunity Plants utilise intracellular nucleotide-binding, leucine-rich repeat (NLR) immune receptors to detect pathogen effectors and activate local and systemic defence. NRG1 and ADR1 “helper” NLRs (RNLs) cooperate with enhanced disease susceptibility 1 (EDS1), senescence-associated gene 101 (SAG101) and phytoalexin-deficient 4 (PAD4) lipase-like proteins to mediate signalling from TIR domain NLR receptors (TNLs). The mechanism of RNL/EDS1 family protein cooperation is not understood. Here, we present genetic and molecular evidence for exclusive EDS1/SAG101/NRG1 and EDS1/PAD4/ADR1 co-functions in TNL immunity. Using immunoprecipitation and mass spectrometry, we show effector recognition-dependent interaction of NRG1 with EDS1 and SAG101, but not PAD4. An EDS1-SAG101 complex interacts with NRG1, and EDS1-PAD4 with ADR1, in an immune-activated state. NRG1 requires an intact nucleotide-binding P-loop motif, and EDS1 a functional EP domain and its partner SAG101, for induced association and immunity. Thus, two distinct modules (NRG1/EDS1/SAG101 and ADR1/EDS1/PAD4) mediate TNL receptor defence signalling. Plants and animals have evolved structurally and functionally related cell surface and intracellular receptors that detect pathogen-derived molecules and activate innate immune responses. In both kingdoms, pathogen recognition by intracellular nucleotide-binding/leucine-rich repeat (NLR) receptors restricts disease [1] . Whereas mammals tend to have few functional NLR receptors, many plants have expanded and diversified NLR gene repertoires, likely in response to evolutionary pressure from host-adapted pathogens and pests [1] , [2] . Despite these different trajectories, plant and mammalian NLRs behave similarly as conformational switches for triggering defence and immune-related death pathways [3] . Plant NLRs directly bind pathogen strain-specific virulence factors (called effectors) or sense their modification of host immunity targets [4] . NLR-effector recognition leads to a process called effector-triggered immunity (ETI) which stops pathogen infection and is often accompanied by localised host cell death [5] . Increasing evidence in mammals and plants suggests NLR activation results from induced NLR oligomerization to form signalling-active scaffolds [6] . Plant NLR receptors are classified on the basis of their N-terminal signalling domain architectures: Toll/interleukin-1 receptor/resistance (TIR) NLRs (or TNLs) and coiled-coil (CC) NLRs (CNLs). The cryo-EM structure of a pathogen-activated CNL pentamer, Arabidopsis ZAR1, shows that five N-terminal domain protomers assemble a putative membrane-associated pore or channel which might represent a CC-mediated mechanism for activating defence signalling [7] . By contrast, structures of two pathogen-activated TNL receptor tetramers, Arabidopsis RPP1 and tobacco ( Nicotiana benthamiana ) Roq1, reveal that the four N-terminal TIR domains become reorganised to create a holoenzyme [8] , [9] . Studies show that TIR-domains have NAD + hydrolysis activity which, for plant TNLs, is necessary to initiate an authentic host immune response [10] , [11] . Hence, CNL- and TNL receptor early outputs appear to be different, though both are initiated by recognition-dependent oligomerization. How NLR activation is transmitted to downstream pathways in ETI is more obscure, although CNLs and TNLs converge on qualitatively similar transcriptional programmes that drive local and systemic resistance [12] , [13] , [14] . NLRs also cooperate with cell surface pattern recognition receptor (PRR) systems mediating pattern-triggered immunity (PTI) to confer a fully effective immune response [15] , [16] . Moreover, CNLs and TNLs rely on a network of signalling NLRs (generically referred to as helper NLRs) to promote immunity and host cell death [17] , [18] , [19] . Two related sub-families of helper NLRs, N requirement gene 1 (NRG1) [20] , [21] and activated disease resistance 1 (ADR1) [22] , are characterised by an N-terminal four-helix bundle domain with homology to Arabidopsis resistance to powdery mildew 8 (RPW8) and plant, fungal and mammalian mixed lineage kinase cell death executors (MLKLs) that have HET-S/LOP-B (HeLo) domains [23] , [24] . These helper NLRs are called CC R -NLRs (or RNLs) [17] . In Arabidopsis , two functionally redundant NRG1 paralogues ( NRG1.1 and NRG1 .2) and three redundant ADR1 paralogues ( ADR1 , ADR1-L1 and ADR1-L2 ) contribute genetically to different extents to resistance and host cell death mediated by CNL and TNL receptors against a range of pathogens [12] , [19] , [25] , [26] . Functionally relevant interactions have not been found so far that would link RNLs molecularly to sensor NLRs or downstream signalling pathways. The enhanced disease susceptibility 1 (EDS1) family of three lipase-like proteins, EDS1, senescence-associated gene 101 (SAG101) and phytoalexin deficient 4 (PAD4), constitutes a major NLR immunity signalling node [27] . EDS1 is essential for TNL-dependent ETI across flowering plant species [26] , [28] , [29] and forms mutually exclusive, functional heterodimers with SAG101 or PAD4 [30] . Genetic and biochemical characterisation of EDS1–SAG101 and EDS1–PAD4 dimers shows they have distinct functions in immunity [26] , [30] , [31] , [32] . EDS1–SAG101 appears to have coevolved with NRG1 group RNLs to signal specifically in TNL-triggered ETI [26] . By contrast, EDS1–PAD4, like ADR1 group RNLs, regulate a basal immunity response which, in Arabidopsis , slows virulent pathogen infection [12] , [22] , [25] , [28] , [32] , [33] and is utilised for ETI by TNL and CNL receptors [12] , [19] , [32] . A major role of EDS1–PAD4 and ADR1 RNLs in Arabidopsis basal immunity is to transcriptionally boost a genetically parallel salicylic acid (SA) phytohormone defence sector, which mediates local and systemic defences and is vulnerable to pathogen effector manipulation [28] , [33] , [34] . Recent studies revealed there is functional cooperation between EDS1–SAG101 and NRG1 RNLs in TNL ETI in Arabidopsis and N. benthamiana , consistent with their co-occurrence in angiosperm species [26] , [29] , [35] . Similarly, Arabidopsis pad4 and adr1 -family mutants phenocopy each other in various ETI and basal immunity responses [25] , [26] . Several groups have proposed that EDS1–SAG101 co-functions with NRG1s, and EDS1–PAD4 with ADR1s, thus constituting two distinct immunity signalling nodes downstream of NLR activation [21] , [25] , [26] . Here we present a genetic and biochemical characterisation of how Arabidopsis NRG1 and ADR1 RNLs co-function with EDS1 family members in NLR-triggered immunity. We show in Arabidopsis that EDS1–SAG101–NRG1 s and EDS1–PAD4–ADR1 s operate genetically as non-interchangeable signalling nodes in ETI. By performing immunoprecipitation and mass spectrometry analyses of Arabidopsis stable transgenic lines, we detect induced specific NRG1 association with EDS1 and SAG101 proteins and ADR1 association with EDS1 and PAD4 after TNL activation. We find in Arabidopsis stable transgenic lines and in N. benthamiana reconstitution assays that PTI activation is insufficient for NRG1-induced association with EDS1 and SAG101. Both the EDS1–SAG101 heterodimer and NRG1 are necessary to form a signalling-active protein complex. Our data provide a molecular insight to two functionally different RNL signalling nodes operating with specific EDS1-family members to mediate defences downstream of NLR receptor activation. Distinct PAD4 - ADR1 and SAG101 – NRG1 modules in TNL RRS1-RPS4 immunity We tested in Arabidopsis whether individual components of the proposed EDS1–PAD4–ADR1 s and EDS1–SAG101–NRG1 s immunity modules [25] , [26] are genetically interchangeable. We reasoned that the replacement of ADR1 by NRG1 group members, and reciprocally PAD4 by SAG101 , would reveal cross-utilization of components. Combinations of previously characterised Arabidopsis EDS1 family mutants ( pad4 , sag101 , and pad4 sag101 ) with ADR1 ( adr1 adr1-L1 adr1-L2 , denoted a3 ) [22] or NRG1 group ( nrg1.1 and nrg1.2 ; denoted n2 [26] ) mutants were generated in accession Col-0 (Col). This produced mutant groups I, II and III (Fig. 1a ), with group III containing between-module combinations. Group I, II and III mutants were tested for resistance mediated by the TNL pair RRS1 and RPS4 (TNL RRS1–RPS4 ) to Pst avrRps4 infection in leaves, measured against wild-type Col-0 (Col, resistant), an rrs1a rrs1b ( rrs1ab ) mutant defective specifically in TNL RRS1–RPS4 ETI [36] , as well as eds1 and an a3 n2 ‘helperless’ mutant which are both fully susceptible to Pst avrRps4 [12] , [19] , [25] , [26] . In Pst avrRps4 bacterial growth assays, pad4 a3 phenocopied the partial resistance of pad4 and a3 single mutants, and sag101 n2 phenocopied sag101 and n2 full resistance (Fig. 1b, c ). The cross-pathway pad4 n2 and sag101 a3 combinations in Group III were as susceptible as eds1 , pad4 sag101 and a3 n2 mutants (Fig. 1b, c ). We further tested group I, II and III mutants for host cell death responses to a type III secretion system-equipped P. fluorescens strain Pf 0-1 delivering avrRps4 , visually at 24 h post infiltration (hpi) (Supplementary Fig. 1a ) and by quantitative electrolyte leakage assays over 6–24 hpi (Supplementary Fig. 1b–e ). This produced the same phenotypic clustering of mutants as the Pst avrRps4 resistance assays— pad4 and a3 behaved like pad4 a3 , while defects in sag101 and n2 aligned with those in sag101 n2 . Put together, these data show that there is exclusive cooperation between PAD4 and ADR1 RNLs in a single pathway leading to restriction of bacterial growth, and between SAG101 and NRG1 RNLs in promoting host cell death and resistance in TNL RRS1–RPS4 immunity. Furthermore, the data argue strongly against physiologically relevant cross-utilization of components between the PAD4–ADR1 s and SAG101–NRG1 s signalling modules. Fig. 1: Distinct PAD4–ADR1 and SAG101–NRG1 modules operate in Arabidopsis TNL RRS1–RPS4 immunity. a Overview of mutants used in ( b ) and ( c ). Group I comprises mutants disabled in SAG101 and/or NRG1 s: sag101 , nrg1.1 nrg1.2 ( n2 ) and sag101 n2 . Group II has mutants in PAD4 and/or ADR1 s: pad4 , adr1 adr1-L1 adr1-L2 ( a3 ) and pad4 a3 . Group III is composed of cross-branch combinatorial mutants a3 n2 , sag101 a3 , pad4 n2 , pad4 sag101 , sag101 pad4 a3 , sag101 pad4 n2 , eds1 pad4 sag101 . b Growth of Pseudomonas syringae pv. tomato DC3000 ( Pst ) avrRps4 in leaves of Arabidopsis Col-0 (Col) and indicated mutants at 3 days post inoculation (dpi) via syringe infiltration (OD 600 = 0.0005). Bacterial loads are shown as log 10 colony-forming units (CFU) per cm 2 . Experiments were performed three times independently with four replicates each (Tukey’s HSD, α = 0.001, n = 12). Error bars represent standard error of mean. Datapoints with the same colour come from one independent experiment. c Growth of Pst avrRps4 , Pst avrRpt2 or Pst (empty vector, EV) in indicated Arabidopsis lines at 3 dpi infected via syringe infiltration (OD 600 = 0.0005). Heatmap represents mean log 10 -transformed CFU values from three ( Pst avrRps4 ), four ( Pst ) or five ( Pst avrRpt2 ) independent experiments, each with four replicates ( n = 12 for Pst avrRps4 , n = 16 for Pst , n = 20 for Pst avrRpt2 ). Statistical significance codes are assigned based on Tukey’s HSD ( α = 0.001). sag101 a3 and pad4 n2 phenocopy pad4 sag101 and a3 n2 , indicating that SAG101 does not form functional signalling modules with ADR1s, and NRG1s with PAD4. Note: significance codes are assigned based on the statistical analysis per treatment and should be read columnwise. The jitter plot in b shows individual data points used to calculate means on the heatmap for Pst avrRps4 infection. Pst Pseudomonas syringae pv. tomato DC3000, CFU colony-forming units, EV empty vector. Full size image The EDS1–SAG101 – NRG1 node is dispensable for CNL RPS2 –dependent ETI Resistance to Pst avrRpt2 mediated by the CNL receptor RPS2 was compromised only when PAD4 or ADR1 RNLs were mutated in group I, II and III mutants, and there was no measurable contribution of SAG101 or NRG1 RNLs to RPS2 immunity, even in a pad4 a3 background (Fig. 1c , Supplementary Fig. 2a ). In quantitative electrolyte leakage assays, we detected equivalent contributions of PAD4 and ADR1 RNLs to RPS2 triggered host cell death at 6 and 8 hpi, but not later at 24 hpi (Supplementary Fig. 3 ), as seen previously for pad4 and eds1 mutants [33] and a3 [12] . Importantly, PAD4 and ADR1 s early promotion of RPS2 cell death could not be substituted by SAG101 or NRG1 s in any of the mutant lines (Supplementary Fig. 3a, b ). We concluded that EDS1-PAD4 also work together with ADR1s in a single pathway to promote CNL RPS2 -triggered early host cell death and that SAG101 and NRG1 s are not recruited for CNL RPS2 ETI, even when PAD4 and ADR1s are disabled. Next, we investigated whether recruitment of PAD4 and ADR1 s and apparent non-utililization of SAG101 and NRG1 s in RPS2-triggered immunity is masked by the genetically parallel ICS1 -dependent SA defence hormone pathway [22] , [32] , [33] , [37] . For this, we introduced an ics1 ( sid2 ) mutation into the single-module ( pad4 a3 , sag101 n2 ) and cross-module ( pad4 n2 and sag101 a3 ) mutant backgrounds (Fig. 2a ). Loss of ICS1 did not alter the different dependencies of TNL RRS1-RPS4 or CNL RPS2 on PAD4–ADR1 s and SAG101–NRG1 s in bacterial resistance (Fig. 2a ; Supplementary Fig. 4a–d ). We concluded that PAD4–ADR1 s and SAG101–NRG1 s distinctive contributions to resistance mediated by these TNL and CNL receptors are independent of ICS1 -generated SA. Fig. 2: Removal of the SAG101–NRG1 and ICS1 sectors reveals PAD4–ADR1 -promoted TNL cell death. a A heatmap representation of Pst avrRps4 , Pst avrRpt2 or Pst (empty vector, EV) growth at 3 dpi in leaves of indicated genotypes (syringe infiltration, OD 600 = 0.0005). The significance codes are based on Tukey’s HSD test ( α = 0.001, n = 12 for Pst avrRps4 and Pst avrRpt2 , n = 16 for Pst ). Data points were combined from three ( Pst avrRps4 , Pst avrRpt2 ) or four ( Pst ) independent experiments, each with four replicates. Note: significance codes are assigned based on the statistical analysis per treatment and should be read columnwise. b A heatmap of quantitative cell death assays conducted on leaves of indicated genotypes after infiltration utilising the Pseudomonas fluorescens 0–1 effector tester strain (hereafter Pf 0-1) delivering avrRps4 (OD 600 = 0.2). Cell death was measured by electrolyte leakage from bacteria-infiltrated leaf discs at 6, 8, 10 and 24 hpi. Data are displayed as means from four experiments, each with four replicates ( n = 16). Statistical significance codes for the difference in means are based on Tukey’s HSD test ( α = 0.001). In mutants marked in red, the PAD4–ADR1 s cell death branch operates in TNL RRS1-RPS4 immunity when SAG101–NRG1 s and ICS1 pathways are not functional. Note: significance codes are assigned based on the statistical analysis per timepoint and should be read columnwise. Boxplot representation of the same data is provided in Supplementary Figs. 5 and 6. c Visual cell death symptoms at 24 hpi Pf 0-1 avrRps4 infiltrating into leaf halves of indicated genotypes as in b . The ratio beneath each leaf indicates number of leaves with visible tissue collapse from all infiltrated leaves in two independent experiments. White arrows mark cell death visible as tissue collapse in a manner dependent on SAG101–NRG1 s. Red arrows mark cell death in lines without functional SAG101–NRG1 s and ICS1 . Genotypes in red have functional PAD4–ADR1s but not SAG101–NRG1 s. Pst Pseudomonas syringae pv. tomato DC3000, Pf 0-1 effector tester strain of Pseudomonas fluorescens 0–1, CFU colony-forming units, EV empty vector. Full size image We further tested whether a possible SAG101 and NRG1 s role in basal resistance against virulent Pst (Fig. 1c , Supplementary Fig. 2b) [12] , [25] is redundant with and therefore obscured by the SA and PAD4 - ADR1 s sectors [13] , [22] , [38] . We found that sag101 and n2 mutations did not increase sid2 , sid2 pad4 and sid2 a3 susceptibility to Pst (Fig. 2a , Supplementary Fig. 4e, f ). Therefore, SAG101 and NRG1 s do not contribute to Arabidopsis basal resistance to Pst bacteria in a susceptible interaction. TNL cell death via PAD4–ADR1 s in the absence of SAG101–NRG1 s and ICS1 SAG101 and NRG1 s are dispensable for TNL RRS1-RPS4 resistance unless PAD4 and/or ADR1 s are disabled (Figs. 1 b, 2a ; Supplementary Fig. 4a, b ), consistent with unequal contributions of these two branches in TNL immunity [12] , [19] , [25] , [26] . We used the Arabidopsis combinatorial mutants with sid2 (Fig. 2a ) to explore whether ICS1- synthesised SA affects PAD4–ADR1 s or SAG101–NRG1 s involvement in TNL RRS1-RPS4 triggered host cell death. In quantitative electrolyte leakage assays over 6–24 hpi and macroscopically at 24 hpi, pad4 , a3 , sid2 , pad4 sid2 and a3 sid2 mutants displayed similar leaf cell death responses as wild-type Col (Fig. 2b, c ; Supplementary Figs. 5 and 6). Therefore, PAD4 and ADR1 s are dispensable for TNL RRS1–RPS4 cell death, regardless of ICS1 -dependent SA status. While n2 and sag101 mutants had strongly reduced host cell death, as expected [12] , [19] , [26] , we observed an early cell death response similar to that of wild-type Col in sag101 sid2 and n2 sid2 backgrounds (Fig. 2b, c ; Supplementary Figs. 5 and 6). This restored cell death was abolished in pad4 sag101 sid2 and a3 n2 sid2 mutants (Fig. 2b, c ; Supplementary Figs. 5 and 6). We concluded that an EDS1–PAD4–ADR1 s controlled mechanism can lead to host cell death in TNL RRS1–RPS4 immunity that is likely antagonised or restricted by combined EDS1–SAG101–NRG1 s and SA functions. Previously, SA was found to conditionally suppress leaf cell death promoted by metacaspase 1 (MC1) in CNL RPM1 ETI [39] , and MC1 , PAD4 or ADR1 s promoted runaway cell death caused by the loss of Lesion Simulating Disease1 ( LSD1 ) [22] , [40] , [41] , [42] . Therefore, we tested whether MC1 is required for the PAD4 –ADR1 s-dependent TNL RRS1–RPS4 cell death that was restored in sag101 sid2 (Fig. 2b, c ; Supplementary Figs. 5 and 6 ). For this, we generated a sag101 sid2 mc1 triple mutant and measured its cell death phenotype alongside mc1 and pad4 sid2 mc1 lines. The mc1 mutation did not compromise SAG101 or PAD4 promoted TNL cell death (Supplementary Fig. 7 ), suggesting that MC1 is dispensable for both SAG101–NRG1 s - and PAD4–ADR1 s-driven cell death responses in TNL-triggered bacterial immunity. Collectively, these data show that EDS1–SAG101–NRG1 s and EDS1–PAD4–ADR1 s are genetically hard-wired signalling modules in NLR immunity that react differently to ICS1 -generated SA. PAD4 and SAG101 interact, respectively, with ADR1s and NRG1s We tested whether the genetic co-requirement of EDS1–PAD4–ADR1 s and EDS1–SAG101–NRG1 s results from specific molecular associations. We generated complementing pPAD4:YFP-PAD4 and pSAG101:SAG101-YFP stable transgenic lines in a Col pad4 sag101 double mutant background (Supplementary Fig. 8 ) to test whether each EDS1 partner associates with similar or different RNL proteins in the TNL ETI response. The double pad4 sag101 mutant background of the pSAG101:SAG101-YFP complementation line allows SAG101–NRG1 s to engage in cell death and pathogen resistance conferred by RRS1–RPS4) [26] (Supplementary Fig. 8 ) and also in transcriptional reprogramming that is otherwise chiefly controlled by PAD4-ADR1 s in TNL RRS1–RPS4 ETI [12] , [32] . These two lines and a Col p35S:YFP-StrepII-3xHA (YFP-SH) control were infiltrated with Pf 0-1 avrRps4 . Pf 0-1 avrRps4 -elicited leaf total soluble extracts were processed at 6 hpi because EDS1 -dependent transcriptional reprogramming starting at ~4 hpi is critical for RRS1–RPS4 resistance [12] , [13] , [32] , [43] . SAG101-YFP, YFP-PAD4 and YFP-SH proteins were purified via immunoprecipitation (IP) with GFP-trap agarose beads. Liquid chromatography and mass spectrometry (MS) (LC–MS) analyses showed strong enrichment of the two Col-0 native EDS1A and EDS1B isoforms in both SAG101-YFP or YFP-PAD4 samples (Fig. 3a ; Supplementary Data 2 ), as expected from earlier studies [30] , [31] , [44] , [45] . EDS1A and EDS1B were also detected at a low level in YFP-SH control IPs (Fig. 3a ), consistent with EDS1 weak non-specific interaction when its direct partners (PAD4 and SAG101) are missing [45] , [46] . NRG1.1 and NRG1.2 peptides were highly enriched in SAG101-YFP but not YFP-PAD4 or YFP-SH samples. Notably, peptides derived from NRG1.3, a truncated NRG1 isoform that does not contribute genetically to TNL ETI responses [25] , were enriched in SAG101-YFP IPs, and less strongly with YFP-PAD4 (Fig. 3a ; Supplementary Fig. 9 ; Supplementary Data 2 ). By contrast, ADR1-L1 and ADR1-L2 co-purified with YFP-PAD4 but were not detected in SAG101-YFP or YFP-SH IP samples (Fig. 3a ; Supplementary Fig. 9 ; Supplementary Data 2 ), suggesting that ADR1 group RNLs interact preferentially with PAD4 over SAG101 at 6 hpi. A number of other immunity components were differentially enriched by SAG101-YFP and PAD4-YFP in the LC–MS analysis (Supplementary Fig. 9b ), consistent with the two EDS1 partners contributing to different processes in TNL RRS1-RPS4 immunity. Put together, the Arabidopsis IP-MS analyses show that EDS1–PAD4 and EDS1–SAG101 dimers interact specifically with RNLs in TNL-induced tissues at 6 hpi. The observed preferential association of PAD4 with ADR1-L1 and ADR1-L2, and SAG101 with NRG1.1 and NRG1.2, further suggests that EDS1–PAD4 and EDS1–SAG101 complexes with specific helper RNL types underpin these genetically distinct Arabidopsis immunity modules promoting host resistance and cell death responses in TNL ETI [19] , [32] (Figs. 1 and 2 ). Fig. 3: Early effector-dependent NRG1 association with EDS1 and SAG101 in Arabidopsis TNL RRS1–RPS4 triggered ETI. a Dotplot of normalised abundance values (label-free quantification (LFQ), log 2 -scaled) for proteins detected in liquid chromatography–mass spectrometry (LC–MS) analyses after α-GFP immunoprecipitation (IP) of PAD4-YFP or SAG101-YFP from total leaf extracts of respective complementation lines pPAD4:YFP-PAD4 and pSAG101:SAG101-YFP (both Col pad4 sag101 background) after infiltration with effector tester stra5in of Pseudomonas fluorescens 0-1 ( Pf 0-1) avrRps4 (6 hpi, OD 600 = 0.2). ADR1s are specifically enriched in PAD4-YFP IP samples, whereas NRG1s are more abundant in the SAG101-YFP IP samples. Samples were collected from four independent experiments. b Dotplot of LFQ values for proteins detected in LC–MS analyses after IP of EDS1-YFP and TRB1-GFP from nuclei-enriched extracts of corresponding Arabidopsis complementation lines infiltrated with Pseudomonas syringae pv. tomato DC3000 ( Pst ) avrRps4 (8 hpi, OD 600 = 0.1). NRG1.1 and NRG1.2 are specifically enriched in EDS1-YFP samples. Samples were collected from four independent experiments. c α-GFP probed immunoblots of nuclei-enriched extracts from leaves of the Arabidopsis pEDS1:EDS1-YFP complementation line (Col eds1-2 background) infiltrated with Pst avrRps4 (OD 600 = 0.1, 8 hpi). Extracts were resolved using native gel filtration. Arrows below protein markers indicate position of the corresponding peak. Numbers refer to column fractions. EDS1 forms stable ~100–600 kDa complexes. The experiment was conducted three times with similar results. d LC–MS analysis of eluates after α-FLAG IP of total leaf extracts from Arabidopsis Ws-2 n2 pNRG1.2:NRG1.2-HF complementation line infiltrated with Pf 0-1 empty vector (EV) or Pf 0-1 avrRps4 (4 hpi, OD 600 = 0.3). Peptides corresponding to EDS1 and SAG101 were observed in eluates only after Pf 0-1-mediated delivery of avrRps4. This result was observed in two independent experiments. e Western blot (WB) analysis of eluates from ( d ). Asterisk indicates a nonspecific band on the α-EDS1 blot for input samples. The analysis was performed on total leaf extracts and was conducted four times with similar results. Association of EDS1 with NRG1.2-HF was observed only after Pf 0-1-mediated delivery of avrRps4. Ponceau S staining shows similar protein loading in input samples on the blot. Full size image Early effector-dependent NRG1 association with EDS1 and SAG101 To investigate whether the RNLs associate with EDS1, we enriched for EDS1 protein from a transgenic Col eds1 line expressing pEDS1:EDS1-YFP [43] at 8 h after infiltrating leaves with Pst avrRps4 bacteria and preparing nuclear-enriched extracts. Garcia et al. (2010) demonstrated the importance of an EDS1 nuclear pool for gene expression reprogramming in TNL RRS1–RPS4 triggered ETI [43] . To interrogate protein associations with EDS1, we immunoprecipitated EDS1-YFP using GFP-trap agarose beads and analysed co-purified proteins via LC–MS. GFP-trap purification and LC–MS processing of eluates from a Col mutant in Telomere Repeat Binding 1 ( TRB1 ) expressing nuclear localised TRB1-GFP [47] was used as a control for non-specific associations (Fig. 3b ; Supplementary Fig. 10 ; Supplementary Data 3 ). PAD4 and SAG101 were highly enriched in EDS1-YFP relative to TRB1-GFP pulldowns, as represented in a volcano plot (Supplementary Fig. 10 ), and consistent with EDS1 stable PAD4 or SAG101 dimers persisting in the TNL RRS1–RPS4 ETI response [44] , [45] . NRG1.1 and NRG1.2 proteins were also specifically enriched in EDS1-YFP compared to TRB1-GFP samples (Fig. 3b ). We did not detect any of the three functional Arabidopsis ADR1 isoforms, ADR1, ADR1-L1 and ADR1-L2 [22] (Fig. 3b ; Supplementary Data 3 ). In the nuclei-enriched protein extracts separated by native size exclusion chromatography, EDS1-YFP eluted between ~50 and ~600 kDa (Fig. 3c ). An EDS1-YFP peak at ~160 kDa with a higher molecular weight tail is consistent with EDS1 forming stable exclusive heterodimers with PAD4 or SAG101 [30] , [31] , [45] and sub-stoichiometric higher-order complexes (Fig. 3c ). Together, these data suggest that NRG1.1 and NRG1.2 also interact with EDS1 in TNL RRS1–RPS4 -activated cells. We tested whether the association of NRG1 group RNLs with EDS1 and SAG101 is dependent on TNL RRS1–RPS4 activation using an Arabidopsis Ws-2 n2 complementation line expressing pNRG1.2:NRG1.2-6xHis-3xFLAG ( NRG1.2-HF ) [19] . Leaves were infiltrated with Pf 0-1 bacteria delivering avrRps4 ( Pf 0-1 avrRps4 ) to activate RRS1–RPS4 ETI or Pf 0-1 with an empty vector (EV) as a negative control eliciting PTI [48] , [49] . Soluble extracts from Pf 0-1 EV and Pf 0-1 avrRps4 -infiltrated leaves at 4 hpi were processed to monitor early changes during the EDS1 -dependent transcriptional reprogramming in TNL RRS1–RPS4 resistance [12] , [13] , [32] , [43] , [49] . After NRG1.2-HF immunopurification on α-FLAG agarose beads, LC–MS analysis revealed spectra for peptides derived from EDS1 and SAG101 in elution products isolated from Pf 0-1 avrRps4 but not Pf 0-1 (EV)-treated tissues (Fig. 3d ). No PAD4 peptides were identified in the analysis (Supplementary Data 4 ). Elution products resolved by SDS–PAGE and probed with α-FLAG and α-EDS1 antibodies also revealed an association of EDS1 with NRG1.2 that is dependent on Pf 0-1 delivery of avrRps4 (Fig. 3e ). Importantly, no association between NRG1.2 and EDS1 or SAG101 was detected at 4 hpi with Pf 0-1 alone, indicating that a PTI response [15] , [16] , [50] is insufficient to induce an NRG1 interaction with EDS1 and SAG101 (Fig. 3d, e ; Supplementary Data 4 ). These data show that TNL RRS1–RPS4 activation induces NRG1.2 associations with EDS1 and SAG101, but not PAD4, in Arabidopsis . NRG1.1 interacts with EDS1 and SAG101 after tobacco TNL activation Previously, transient co-expression of Arabidopsis EDS1, SAG101 and NRG1.1 or NRG1.2 proteins in an N. benthamiana CRISPR quadruple eds1a pad4 sag101a sag101b ( Nb epss ) mutant reconstituted host cell death and bacterial resistance after TNL Roq1 recognition of the bacterial effector XopQ [26] , [51] . We exploited the Nb epss transient assay system to investigate molecular requirements for Arabidopsis EDS1, SAG101, NRG1s associations and functions in ETI. For this, we developed an ETI assay in Nb epss leaves with more precise timing of the TNL Roq1 -dependent response than previously achieved using only Agrobacteria -mediated expression of various components [26] . In the modified assay, we transiently expressed combinations of epitope-tagged proteins in Nb epss leaf zones using Agrobacteria and, after 48 h, infiltrated Pf 0-1 XopQ bacteria to activate TNL Roq1 immunity (Fig. 4a ). Co-expression of Arabidopsis EDS1-FLAG, SAG101-FLAG and NRG1.1-SH led to XopQ-dependent host cell death quantified in electrolyte leakage assays at 24 hpi (Fig. 4b ). In this ETI assay, replacement of Arabidopsis NRG1.1-SH by ADR1-L2-SH or co-expression of GUS-FLAG with NRG1.1-SH did not lead to XopQ-triggered host cell death (Fig. 4b ), consistent with PAD4 being dispensable for TNL immune responses in N. benthamiana [26] , [29] , even with a Pf 0-1 stimulus. Fig. 4: XopQ/Roq1-dependent Arabidopsis NRG1.1 association with EDS1 and SAG101 in Nicotiana benthamiana . a Sample collection scheme for experiments in ( b ) and ( c ). Roq1-dependent cell death is restored in Nicotiana benthamiana ( Nb ) eds1 pad4 sag101a sag101b ( Nb epss ) signalling deficient mutant by expressing Arabidopsis EDS1, SAG101 and NRG1.1 via Agrobacteria infiltration 48 h before XopQ effector delivery. Pf 0-1 XopQ is syringe-infiltrated (OD 600 = 0.3) to deliver the effector and to study TNL signalling events in a time-resolved manner up to 24 hpi. b Macroscopic symptoms and quantification of XopQ-triggered cell death at 24 hpi after infiltrating Pf 0-1 XopQ in leaves of Nb epss expressing Arabidopsis EDS1-FLAG, SAG101-FLAG, NRG1.1-3xHA-StrepII (NRG1.1-SH) or ADR1-L2-3xHA-StrepII (ADR1-L2-SH). Pf 0-1 with empty vector ( Pf 0-1) served as a “no-ETI” control. Cell death was quantified in electrolyte leakage assays 6 h after harvesting leaf discs (24 hpi with Pf 0-1 XopQ ). The experiment was performed three times independently, each with four replicates (leaf discs) (Tukey’s HSD, α = 0.001, n = 12). Transiently expressed Arabidopsis EDS1, SAG101 and NRG1.1 proteins are functional in Pf 0-1 XopQ triggered (Roq1) cell death. Description of boxplots: minima—first quartile, maxima—third quartile, centre—median, whiskers extend to the minimum and maximum values but not further than 1.5 interquartile range from the respective minima or maxima of the boxplot. Datapoints with the same colour come from one independent experiment. c Coimmunoprecipitation assay followed by Western blotting to test for XopQ-triggered associations between Arabidopsis NRG1.1-SH and FLAG-tagged EDS1 or SAG101 in Nb epss according to the infiltration scheme in ( a ). NRG1.1-SH or ADR1-SH were enriched using α-HA agarose beads, and presence of FLAG-tagged EDS1, SAG101 or GUS was tested by probing blots with α-FLAG antibodies. IP assays were conducted three times independently with similar results. NRG1.1 association with EDS1 and SAG101 requires Roq1/XopQ ETI activation. Pf 0-1 effector tester strain of Pseudomonas fluorescens 0–1 with empty vector, Pf 0-1 XopQ (in a ) or XopQ ( Pf 0-1) effector tester strain of Pseudomonas fluorescens 0–1 delivering XopQ , WB Western blotting, IP immunoprecipitation, Nb epss Nicotiana benthamiana eds1a pad4 sag101a sag101b . Full size image We performed a time course to monitor the accumulation and associations of NRG1.1-SH with EDS1-FLAG and SAG101-FLAG in Nb epss leaf samples harvested at 4, 8, 12 and 24 h after Pf 0-1 XopQ inoculation. Although protein inputs were similar in all samples, a clear NRG1.1–SAG101 and NRG1.1–EDS1 interaction was detected in α-HA immunopurified samples only at 8 and 12 hpi with Pf 0-1 XopQ (Fig. 4c ). The immunoprecipitation (IP) signals were no longer detectable at 24 hpi, suggesting that Roq1 recognition of Pf 0-1 XopQ -induced NRG1 association with EDS1 and SAG101 is transient and/or disrupted by host cell death at 24 hpi (Fig. 4b, c ). As in Arabidopsis , no association between NRG1.1 and EDS1 or SAG101 was detected at 12 hpi with Pf 0-1 alone (Fig. 4c ), further indicating that a PTI response in N. benthamiana is insufficient to induce NRG1 association with EDS1 and SAG101. Similarly, when Arabidopsis ADR1-L2-SH was expressed instead of NRG1.1-SH in the Nb epss TNL Roq1 ETI assay, it did not interact with SAG101-FLAG or EDS1-FLAG at 12 hpi (Fig. 4c ), mirroring the failure of ADR1-L2 to signal Roq1-triggered host cell death or bacterial resistance in N. benthamiana (Fig. 4b ) [26] . These data show that XopQ activation of TNL Roq1 in Nb epss leaves is necessary to induce NRG1.1 interaction with SAG101 and EDS1 proteins from Arabidopsis . The similarity between Arabidopsis EDS1 family protein associations with RNLs observed in native Arabidopsis (Fig. 3 ) and non-native N. benthamiana (Fig. 4 ) suggests that interaction specificity determines function of the Arabidopsis EDS1 - SAG101 - NRG1 s module in TNL immunity. Analyses in both systems also show that a PTI stimulus alone does not promote NRG1 association with EDS1 and SAG101. EDS1 EP domain-dependent NRG1 association with EDS1 and SAG101 Assembly of Arabidopsis EDS1 heterodimers with PAD4 or SAG101 is mediated by a short N-terminal EDS1 α-helix (αH) fitting into an N-terminal hydrophobic groove of either partner [30] , [32] , [46] . Protein structure–function studies of Arabidopsis and tomato EDS1–SAG101 complexes showed that the heterodimer brings into close proximity two α-helical coils (EDS1 αP and SAG101 αN) on the partner C-terminal ‘EP’ domains, which are essential for TNL ETI signalling [26] , [29] , [30] , [32] . Arabidopsis EDS1 residues F419 and H476 are positioned close to SAG101 αN in the dimer cavity (Fig. 5a ) [26] . In earlier Agrobacteria -only based Nb epss reconstitution assays, an Arabidopsis EDS1 F419E mutation disabled TNL Roq1 signalling without disrupting the EDS1-SAG101 heterodimer [26] . In the Agrobacteria plus Pf 0 - 1 XopQ TNL Roq1 assay (Fig. 4a ), Arabidopsis EDS1 F419E -FLAG and EDS1 H476Y -FLAG single amino acid exchange variants failed to mediate XopQ/Roq1-dependent host leaf cell death at 24 hpi or Xanthomonas euvesicatoria (formerly, Xanthomonas campestris pv. vesicatoria , Xcv ) growth at 6 dpi (Fig. 5b, c ). Also, substituting NRG1.1-SH with ADR1-L2-SH did not confer TNL Roq1 -triggered host cell death and Xcv resistance (Fig. 5b, c ). We monitored the expression of FLAG-tagged EDS1 family proteins by immunoblotting and performed NRG1.1-SH α-HA IP assays on Pf 0-1 XopQ -triggered leaf protein extracts at 10–12 hpi when TNL-induced NRG1.1–EDS1 and NRG1.1–SAG101 associations were strongest (Fig. 4c ). As negative controls, PAD4-FLAG was substituted for SAG101-FLAG, GUS-FLAG for EDS1-FLAG, and ADR-L2-SH for NRG1.1-SH (Fig. 5d ). While all proteins were detected in input samples, NRG1.1 was detected only when NRG1.1-SH was co-expressed together with functional wild-type EDS1-FLAG and SAG101-FLAG (Fig. 5d ). The failure of NRG1.1 to IP SAG101 with GUS replacing EDS1 (Fig. 5d ), indicates that NRG1.1 associates specifically with the EDS1–SAG101 heterodimer and not individual EDS1 or SAG101 monomers, upon triggering of TNL Roq1 ETI. The strong reduction in NRG1.1 association with EDS1 EP domain non-functional variants EDS1 F419E or EDS1 H476Y shows that NRG1 fails to associate with a signalling-inactive EDS1–SAG101 heterodimer after Roq1 activation. Fig. 5: Effector-dependent NRG1–EDS1–SAG101 association requires a functional EDS1 EP domain. a The Arabidopsis EDS1 (green)—SAG101 (purple) heterodimer crystal structure (PDB: 4NFU) with highlighted EP domain cavity essential for TNL-triggered cell death. An α-helix of the SAG101 EP domain (blue) and residues F419 (magenta) and H476 (orange) in EDS1 EP domain are shown as ribbon and spheres, respectively. b , c Roq1/XopQ-dependent cell death ( b ) and bacterial Xcv resistance ( c ) in leaves of Nb epss transiently expressing of C-terminally FLAG-tagged EDS1 wildtype and mutant variants with SAG101-FLAG and NRG1.1-SH or ADR1-L2-SH. Cell death was triggered by infiltrating Pf 0-1 XopQ at 48 h after Agrobacteria infiltration; photos of leaves were taken at 24 h. F419E and H476Y mutations in the Arabidopsis EDS1 EP domain abrogated cell death and resistance. Experiments were performed three times independently, each with four replicates (leaf discs) (Tukey’s HSD, α = 0.001, n = 12). Error bars represent standard error of mean. Description of boxplots: minima—first quartile, maxima—third quartile, centre—median, whiskers extend to the minimum and maximum values but not further than 1.5 inter-quartile range from respective minima or maxima of the boxplot. Datapoints with the same colour come from one independent experiment. d IP followed by Western blot analysis to test the dependency of associations between Arabidopsis EDS1, SAG101 and NRG1.1 in Nb epss on a functional EDS1 EP domain cavity. Leaves of Nb epss were infiltrated with Agrobacteria to express FLAG-tagged EDS1 or its variants EDS1 F419E and EDS1 H476Y , SAG101-FLAG and NRG1.1-SH or PAD4-FLAG, with ADR1-L2-SH and GUS-FLAG as negative controls. At 2 dpi, Pf 0-1 XopQ (OD 600 = 0.3) was infiltrated, and the triggered samples were collected at 10 hpi. Following IP with α-HA agarose beads, input and IP fractions were probed with α-HA and α-FLAG antibodies. Roq1/XopQ-dependent association of NRG1.1-SH with EDS1-FLAG and SAG101-FLAG was abolished in samples with mutated EDS1 EP domain variants. Similar results were obtained in three independent experiments. Xcv Xanthomonas campestris pv. vesicatoria strain 85-10, XopQ ( Pf 0-1) effector tester strain of Pseudomonas fluorescens 0–1 delivering XopQ, WB Western blotting, IP immunoprecipitation, Nb epss Nicotiana benthamiana eds1a pad4 sag101a sag101b . Full size image EDS1 and SAG101 signalling requires an intact NRG1 P-loop and N-terminus We next examined NRG1 molecular features that might influence its TNL signalling function and association with EDS1–SAG101. Because RNLs have domain architectures similar to sensor CNL proteins [17] , we modelled NRG1.1 onto the cryo-EM structure of the activated Arabidopsis CNL receptor ZAR1 which forms a pentameric resistosome [7] . The ZAR1 signalling active pentamer has five exposed N-terminal α-helices (α1) preceding the CC domains of the NLR protomers, which assemble into a potential membrane-associated pore or channel [7] . Structural modelling of Arabidopsis NRG1.1 identified two negatively charged N-terminal glutamic acid (E) residues (E14 and E27) (Fig. 6a ) positioned similarly to ZAR1 α1-helix residues E11 and E18 that are part of the ZAR1 inner funnel and are necessary for ZAR1 resistosome activity [7] . Two other NRG1.1 N-terminal residues, leucine 21 (L21) and lysine 22 (K22) (Fig. 6a ), aligned with L10 and L14 in the ZAR1 α1-helix which promoted ZAR1 membrane association and resistosome signalling [7] . Neither set of ZAR1 α1-helix amino acids was required for effector-induced pentamer assembly [7] . We further identified in Arabidopsis NRG1 RNLs the conserved NLR nucleotide-binding domain (NBD) P-loop (GxxxxGK(T/S)) motif (G 199 K 200 T 201 in Arabidopsis At NRG1.1; Fig. 6a ; Supplementary Fig. 11 ), which mediates nucleotide binding [52] , [53] , and induced self-association and/or signalling functions of several sensor NLRs [54] , [55] . The P-loop was reported to be dispensable for ADR1-L2 conferred resistance during ETI and basal immunity and NRG1.1-conditioned TNL chs3-2D auto-immunity [22] , [25] , but was required for ADR1-L2-conditioned lsd1 -mediated cell death and NRG1 -dependent TNL Roq1 immunity [35] , [41] . Fig. 6: Association between Arabidopsis NRG1.1, EDS1 and SAG101 require an intact NRG1.1 P-loop. a A structure homology model of Arabidopsis NRG1.1 based on the ZAR1 resistosome. NRG1.1 amino acids E14 and E27 (red sticks) and L21 and K22 (blue sticks) aligned with residues E11, E18, F9, L10 and L14 in ZAR1. The modelled NRG1.1 P-loop motif (G199 K200 T201) is shown as cyan sticks. XopQ-triggered cell death ( b ) and Xanthomonas campestris pv. vesicatoria strain 85-10 ( Xcv ) growth restriction ( c ) in Nicotiana benthamiana eds1a pad4 sag101a sag101b ( Nb epss ) expressing Arabidopsis NRG1.1-SH wildtype, NRG1.1 E14A/E27A , NRG1.1 L21A/K22A and NRG1.1 G199A/K200A/T201A variants together with EDS1-FLAG and SAG101-FLAG. Arabidopsis proteins were expressed via Agrobacteria -mediated transient expression assays two days before infiltration of Pseudomonas fluorescens 0-1 ( Pf 0-1) XopQ (OD 600 = 0.3) or simultaneously with Xcv (OD 600 = 0.0005). Experiments were performed three times independently, each with four replicates (leaf discs) (Tukey’s HSD, α = 0.001, n = 12). Error bars represent standard error of mean. Datapoints with the same colour come from one independent experiment. d Immunoprecipitation (IP) and Western blot (WB) analyses testing associations of Arabidopsis NRG1.1 mutant variants with EDS1 and SAG101 in Nb epss after triggering Roq1 signalling by Pf 0-1 XopQ infiltration (OD 600 = 0.3; 10 hpi). Arabidopsis EDS1-FLAG, SAG101-FLAG with NRG1.1-SH, and using GUS-FLAG and Arabidopsis ADR1-L2-SH as negative controls, were expressed using Agrobacteria 2 d prior to Pf 0-1 XopQ infiltration. After α-HA IP, the indicated fractions were analysed with α-HA and α-FLAG antibodies by WB. The experiment was conducted three times independently with similar results. e Model of molecular events leading to generation of an Arabidopsis EDS1–SAG101–NRG1 signalling complex essential for TNL receptor-activated defence. NRG1–EDS1–SAG101 association is dependent on TNL activation and requires an intact EDS1–SAG101 heterodimer EP domain cavity (purple circle) and NRG1 nucleotide-binding domain. In two depicted scenarios, an effector-induced TNL oligomer with NADase activity leads to activation (asterisks) of EDS1–SAG101 via the EP domain cavity (‘Path A’, asterisk inside the purple circle) or NRG1 (‘Path B’). These paths are not mutually exclusive. EDS1–SAG101–NRG1 assembly precedes and is necessary for TNL-triggered cell death and resistance involving a predicted NRG1 N-terminal HeLo domain α-helix. Full size image We made amino acid exchanges to alanines in the NRG1.1 predicted α1-helix E11/E27 (denoted EE) and L21/K22 (LK) pairs and a non-functional NRG1.1 G 199 K 200 T 201 /AAA P-loop variant (denoted GKT). When co-expressed with Arabidopsis EDS1 and SAG101 in the Nb epss TNL Roq1 assay, NRG1.1 EE and NRG1.1 GKT variants were non-functional and NRG1.1 LK was partially functional in eliciting host cell death (Fig. 6b ). All mutant NRG1.1-HA variants failed to confer Xcv resistance (Fig. 6c ). The NRG1.1-HA variants were detected on immunoblots, as were co-expressed EDS1-FLAG and SAG101-FLAG proteins (Fig. 6d ; left panel). In NRG1.1 α-HA IP assays, the NRG1.1-HA N-terminal EE and LK mutants immunoprecipitated EDS1-FLAG and SAG101-FLAG as efficiently as wild-type NRG1.1-SH (Fig. 6d ; right panel). By contrast, the NRG1.1 P-loop GKT mutant displayed a much weaker association with EDS1 and SAG101 (Fig. 6d ; right panel). Failure of NRG1.1 GKT to interact with EDS1 and SAG101 indicates a requirement for ADP/ATP binding and/or nucleotide exchange at the NRG1.1 nucleotide-binding domain for TNL-induced association with EDS1–SAG101 and immunity. Retention of NRG1.1 EE and NRG1.1 LK TNL induced association with EDS1–SAG101, but their loss of immunity activity, suggests that an intact NRG1.1 N-terminal putative α-helix is required for NRG1 signalling in TNL ETI as part of or after its TNL-induced association with EDS1–SAG101. Plant intracellular NLR receptors, activated directly or indirectly by pathogen effectors, provide a critical surveillance mechanism against disease. Activated forms of the two major sensor NLR classes, TNLs and CNLs, assemble into oligomers that are required for immunity signalling and broadly resemble mammalian NLR inflammasome scaffolds [7] , [8] , [9] , [56] . Two phylogenetically related groups of HeLo domain helper NLRs (NRG1s and ADR1s) and the EDS1 family of plant-specific lipase-like proteins (EDS1, PAD4 and SAG101) mediate signalling downstream of sensor NLRs, leading to transcriptional defences and localised host cell death [19] , [25] , [26] , [28] , [35] . Here we provide genetic and molecular evidence in Arabidopsis that distinct RNL immunity modules (or branches) operate with specific EDS1 family heterodimers. The two modules contribute in different ways to TNL RRS1–RPS4 and CNL RPS2 ETI, and to basal immunity against virulent bacteria (Figs. 1 and 2 ; Supplementary Figs. 1 – 6 ). We show in Arabidopsis and N. benthamiana that TNL-effector activation induces a specific association between NRG1 proteins and EDS1–SAG101 heterodimers (Figs. 3 and 4 ). In N. benthamiana TNL Roq1 ETI reconstitution assays, interactions of NRG1 with EDS1 and SAG101 and effective TNL immunity signalling require a functional EDS1 EP domain within the EDS1–SAG101 heterodimer and an intact P-loop motif in NRG1 for nucleotide binding (Figs. 5 and 6 ). Conserved amino acids at the NRG1 N-terminus, modelled onto the structure of a CNL receptor (ZAR1) membrane pore-forming α1-helix [7] , are important for TNL ETI but not for TNL-induced NRG1 association with EDS1–SAG101 (Fig. 6 ). Our data provide a molecular underpinning for genetically separate RNL-EDS1 mechanisms conferring immunity and cell death downstream of NLR-mediated effector recognition (Figs. 1 and 2 ) [25] , [26] , [28] . The data also suggest that sensor NLR-induced assembly of helper NLRs with EDS1 family proteins is a critical step in TNL downstream signalling. Previous studies in Arabidopsis revealed unequal genetic and transcriptional contributions (unequal redundancy) of PAD4 vs. SAG101 [19] , [25] , [26] , [31] and ADR1 vs. NRG1 groups in ETI and basal immunity responses to pathogens [12] , [26] . Arabidopsis SAG101 and NRG1 s function in ETI mediated by TNL receptors and are drivers of TNL host cell death and transcriptional reprogramming [12] , [26] , [27] . PAD4 and ADR1 s are recruited more broadly for TNL and CNL ETI immune responses, in which they control transcriptional SA-dependent and SA-independent defence pathways [22] , [28] , [32] , [33] . Our analysis of Arabidopsis pad4, sag101, adr1- and nrg1 -group combinatorial mutants shows that individual components of the two immunity modules are not interchangeable in TNL RRS1-RPS4 or CNL RPS2 immune responses. These data reveal a specificity in module composition and function (Fig. 1 ; Supplementary Figs. 1 – 3 ). Removing the ICS1- dependent SA pathway uncovered the extent to which separate PAD4 - ADR1 s and SAG101 - NRG1 s genetic mechanisms are preserved (Fig. 2 ; Supplementary Figs. 5 and 6 ). The SA pathway is bolstered in Arabidopsis by PAD4 and ADR1 s via a mutually reinforcing feedback loop [22] , [33] , [41] , [57] . Notably, the removal of ICS1 and SAG101 together, released a PAD4 - ADR1 s activity leading to host cell death in TNL RRS1–RPS4 immunity (Fig. 2b, c ). Hence, each TNL signalling branch has a transcriptional reprogramming and cell death-inducing capacity, depending on the status of other pathways in the network [5] , [58] , [59] . SAG101-NRG1 s and SA antagonism of PAD4-ADR1 s-stimulated cell death suggests there is crosstalk between the different sectors, possibly to limit host tissue damage and promote systemic relay of immunity signals [28] . This aligns with a reported role of SA receptor non-expressor of PR1 (NPR1) in limiting NLR cell death in the presence of high SA concentrations around the tissue undergoing cell death [60] . Although metacaspase 1 (MC1) controlled proteolysis promoting RPM1 cell death is also conditionally antagonised by SA [39] , we did not detect a role for MC1 in SAG101-NRG1 s or PAD4 - ADR1 s stimulated TNL RRS1–RPS4 triggered cell death (Supplementary Fig. 7 ). Arabidopsis IP–LC–MS analyses using EDS1, SAG101, PAD4 and NRG1.2 individually as baits were performed in TNL RRS1–RPS4 triggered leaf tissues between 4 and 8 h after bacterial infiltration, based on knowledge of a critical 4–8 h time window needed for EDS1-PAD4 and ADR1s mobilised gene expression to be effective in immunity [12] , [13] , [32] , [43] , [49] . Also, Arabidopsis TNL RRS1–RPS4 triggered SAG101-NRG1 s-dependent cell death started to increase from 6–8 hpi with Pf 0-1 avrRps4 (Fig. 2 ; Supplementary Fig. 1 ) [26] . The sum of IP–MS data (Fig. 3 ) points to molecular specificity in EDS1–SAG101 interaction with NRG1.1 and NRG1.2 functional isoforms, and in EDS1–PAD4 interaction with ADR1-L1 and ADR-L2 isoforms, in TNL receptor-induced cells. The dynamics of EDS1–SAG101–NRG1s associations relative to presumed EDS1–PAD4–ADR1s associations in immune-activated cells and tissues remain unresolved. The absence of a detectable association between NRG1.2 with EDS1 or SAG101 at 4 h after Pf 0-1 EV treatment (Fig. 3d ), shows that PTI alone is insufficient to induce an NRG1 interaction with EDS1 or SAG101. These data imply that NRG1.2 association with EDS1 and SAG101 requires an activated TNL-derived signal. We suggest it is likely that an EDS1–SAG101–NRG1 functional interaction is principally a post-transcriptional event because (i) it was detected in Arabidopsis at 4 hpi (Fig. 3d, e ) before the main EDS1 -dependent transcriptional elevation at 8–10 hpi [12] , [32] , [49] and (ii) it could be recapitulated in N. benthamiana with abundant transiently expressed proteins only after an effector-TNL trigger (Fig. 4c ). Although we detected a specific association between PAD4 and ADR1s in TNL immune-activated Arabidopsis tissues (Fig. 3 ; Supplementary Fig. 9 ; Supplementary Data 2 ), it has yet to be determined whether their interaction is dependent on a PTI and/or ETI trigger. The preferential enrichment of several cell surface PTI-related proteins by PAD4 in TNL-triggered Arabidopsis tissues (Supplementary Fig. 9 ) is consistent with the EDS1-PAD4-ADR1 node contributing to proposed connectivity between ETI and PTI responses [15] , [16] , [61] . Interestingly, signalling inactive truncated NRG1.3 isoform [25] was enriched with SAG101 and to a lesser extent with PAD4 (Fig. 3a ; Supplementary Fig. 9b ). This might reflect an NRG1.3 role in the negative regulation of both modules. Indeed, Arabidopsis NRG1.3 appears to interfere with the defence signalling by NRG1.1 and NRG1.2 [62] . It is also possible that NRG1 determinants for preferential association with EDS1–SAG101 lie in the NRG1 C-terminal portion. Weak association detected between PAD4 and NRG1.1 (Fig. 5d ) also deviates from otherwise clear-cut specific interactions of within-module components (Fig. 3a ). However, these associations are unlikely to contribute to Arabidopsis TNL immune signalling (Fig. 1 ) [26] . We interrogated the molecular requirements for Arabidopsis EDS1 and SAG101 functional association with NRG1.1 in Nb epss TNL Roq1 transient reconstitution assays. TNL ETI-induced NRG1.1 association was only observed in IPs with EDS1 and SAG101 together (Figs. 4 c, 5 d, 6d ), supporting NRG1 interaction with a signalling competent EDS1–SAG101 heterodimer (Fig. 3 ) but not with EDS1 or SAG101 individually (Fig. 5d ) which are inactive [30] , [45] , [46] . A previous study proposed that NRG1 signals downstream of EDS1 in regulating TNL Roq1 immunity and cell death [35] . Our protein interaction assays instead point to NRG1 working biochemically together with EDS1–SAG101 in the TNL Roq1 immunity signalling cascade, although we cannot exclude NRG1 subsequently dissociating from an EDS1–SAG101 complex as part of the immune response. The discrete timing of NRG1–EDS1–SAG101 interaction detection between 8 and 12 hpi suggests it is transient in nature, although it is unclear in this system whether reduced association at later time-points is a controlled event, possibly to dampen outputs, or due to cell death. A requirement for EDS1 EP-domain essential residues within the EDS1–SAG101 heterodimer [26] , [29] to interact with NRG1.1 in a TNL ETI-dependent manner (Fig. 5d ), suggests that an intact EDS1–SAG101 EP-domain drives its association with NRG1 downstream of TNL receptor activation, as depicted in a model (Fig. 6e ). TNL-induced NRG1–EDS1–SAG101 association and ETI also required a nucleotide-binding form of NRG1.1, whereas N-terminal NRG1.1 amino acids on a ZAR1-like functional N-terminal α-helix, were dispensable for their association (Fig. 6d ). Together, these data argue for TNL effector recognition rendering both NRG1 and EDS1–SAG101 competent to interact and confer pathogen resistance (Fig. 6e ). Recently, the TIR domains of plant TNLs and certain truncated TIR forms were shown to exhibit an NADase activity (shown in Fig. 6e ) that is necessary to induce plant EDS1 -dependent cell death [10] , [11] , [63] . Reported cryo-EM structures of effector-activated TNLs Arabidopsis RPP1 and N. benthamiana Roq1 reveal them to be tetrameric complexes with imposed TIR domain orientations creating an active NADase enzyme [8] , [9] . Our findings suggest concerted actions between plant TNL NADase activity and immunity signalling via TNL-effector recognition induced EDS1–SAG101–NRG1 association. In our model (Fig. 6e ), we envisage two paths for generating a signalling competent NRG1–EDS1–SAG101 complex. In path A, a TNL-derived NADase product binds to EDS1–SAG101, thereby enabling EP domain-dependent association with NRG1, perhaps promoting NRG1 oligomerization. In path B, the activated TNL receptor and/or NADase products cause an NRG1 nucleotide-dependent conformational change (independently of EDS1–SAG101) which promotes its association with EDS1–SAG101. The data presented here represent a significant advance by showing that pathogen-activated TNL receptors mediate downstream signalling via induced, specific interactions between RNLs and EDS1 family proteins. Plant materials and growth conditions Arabidopsis thaliana L. Heynh. 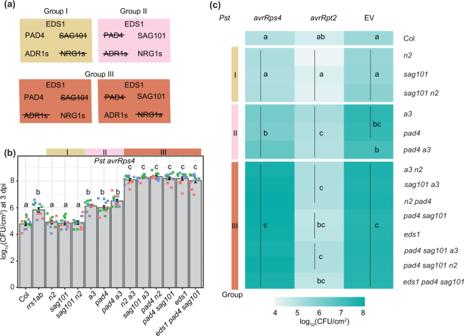Fig. 1: DistinctPAD4–ADR1andSAG101–NRG1modules operate inArabidopsisTNLRRS1–RPS4immunity. aOverview of mutants used in (b) and (c). Group I comprises mutants disabled inSAG101and/orNRG1s:sag101,nrg1.1 nrg1.2(n2) andsag101 n2. Group II has mutants inPAD4and/orADR1s:pad4,adr1 adr1-L1 adr1-L2(a3) andpad4 a3. Group III is composed of cross-branch combinatorial mutantsa3 n2,sag101 a3,pad4 n2,pad4 sag101,sag101 pad4 a3,sag101 pad4 n2,eds1 pad4 sag101.bGrowth ofPseudomonas syringaepv.tomatoDC3000 (Pst)avrRps4in leaves ofArabidopsisCol-0 (Col) and indicated mutants at 3 days post inoculation (dpi) via syringe infiltration (OD600= 0.0005). Bacterial loads are shown as log10colony-forming units (CFU) per cm2. Experiments were performed three times independently with four replicates each (Tukey’s HSD,α= 0.001,n= 12). Error bars represent standard error of mean. Datapoints with the same colour come from one independent experiment.cGrowth ofPst avrRps4,Pst avrRpt2orPst(empty vector, EV) in indicatedArabidopsislines at 3 dpi infected via syringe infiltration (OD600= 0.0005). Heatmap represents mean log10-transformed CFU values from three (Pst avrRps4), four (Pst) or five (Pst avrRpt2) independent experiments, each with four replicates (n= 12 forPst avrRps4,n= 16 forPst,n= 20 forPst avrRpt2). Statistical significance codes are assigned based on Tukey’s HSD (α= 0.001).sag101 a3andpad4 n2phenocopypad4 sag101anda3 n2, indicating that SAG101 does not form functional signalling modules with ADR1s, and NRG1s with PAD4. Note: significance codes are assigned based on the statistical analysis per treatment and should be read columnwise. The jitter plot inbshows individual data points used to calculate means on the heatmap forPst avrRps4infection.PstPseudomonas syringaepv.tomatoDC3000, CFU colony-forming units, EV empty vector. (hereafter Arabidopsis ) wild type, transgenic and mutant lines as well as N. benthamiana lines are listed in Supplementary Table 1 . For pathogen growth and cell death assays, Arabidopsis plants were grown under short-day conditions (10 h light 22 °C/14 h dark 20 °C, light intensity of ~100 μmol m −2 s −1 , 65% relative humidity) for 4–5 weeks. Crosses and seed propagation were conducted under speed breeding growth conditions: 22 h light 22 °C/2 h dark 20 °C, ~100 μmol m −2 s −1 , 65% relative humidity. N. benthamiana plants were grown in a greenhouse under long-day conditions for 5–6 weeks. Cloning and generation of complementation lines Genomic Col-0 SAG101 sequence (AT5G14930.2) including the coding and upstream (−992 bp) sequences were cloned into pENTR/D-TOPO (K240020, Thermo Fisher Scientific) and further LR-inserted (11791100, Thermo Fisher Scientific) into the expression vector pXCG-mYFP [63] resulting in pXCG pSAG101:SAG101-YFP. pXCSG p35S:NRG1.1-StrepII-3xHA as well as the pXCSG pADR1-L2:ADR1-L2-StrepII-3xHA constructs were described previously [26] . Constructs to express NRG1.1 mutant variants were prepared using the Golden gate MolClo kit [64] . The genomic sequence of Col-0 NRG1.1 (AT5G66900.1, from start ATG codon to the last codon position) was cloned into the level 0 plasmid pAGM1287, and the NRG1.1 variants were generated following the QuikChange II Site-Directed mutagenesis (SDM) protocol (#200555, Agilent). Level 0 golden gate compatible construct for the genomic sequence of Col-0 EDS1 (AT3G48090.1, from the first to the last codon) was synthesised and inserted into the pAM vector (GeneArt, Thermo Fisher Scientific). EDS1 H476Y and EDS1 F419E mutant constructs were generated via SDM. Primers for cloning and SDM are listed in Supplementary Data 1 . To obtain level 1 expression constructs, level 0 constructs of NRG1.1 mutants were combined with the cauliflower mosaic virus (CaMV) 35S promoter (pICH51288), hemagglutinin tag (3xHA, pICSL50009), CaMV 35S terminator (pICH41414) and the backbone pICH47732. Expression vectors for EDS1 (p35S:EDS1 H476Y -3xFLAG, p35S:EDS1 F419E -3xFLAG) were cloned following the same strategy except the tag module was replaced by 3xFLAG (pICSL50007). The wild type p35S:EDS1-3xFLAG was prepared by LR-recombining pENTR/D-TOPO EDS1_noStop (genomic sequence of AT3G48090.1 from ATG to the last codon [30] with pAMPAT-3xFLAG [64] . p35S:PAD4-3xFLAG expression construct is a result of a LR reaction between pENTR/D-TOPO PAD4 [30] and pAMPAT-3xFLAG. p35S:3xFLAG-GUS was prepared by LR-recombining pJ2B-3xFLAG [64] with pENTR GUS (from LR clonase II kit, 11791020, Thermo Fisher Scientific). To prepare the PAD4 expression construct for complementation, we PCR-amplified the PAD4 locus (AT3G52430.1) from the upstream gene’s stop codon (AT3G52420) up to the start codon of the downstream gene (AT3G52440) and placed it in a pDONR201 vector via PIPE-PCR [65] . Subsequently, N-terminal YFP with a linker peptide (Gly followed by 9x Ala) was introduced via PIPE-PCR as well. This construct was LR-recombined in a pAlligator2 destination vector [66] . 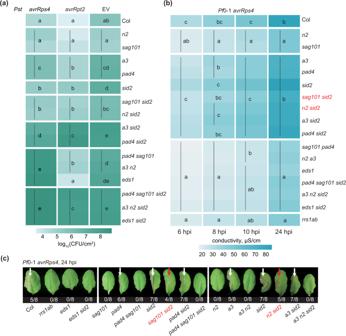Fig. 2: Removal of theSAG101–NRG1andICS1sectors revealsPAD4–ADR1-promoted TNL cell death. aA heatmap representation ofPst avrRps4,Pst avrRpt2orPst(empty vector, EV) growth at 3 dpi in leaves of indicated genotypes (syringe infiltration, OD600= 0.0005). The significance codes are based on Tukey’s HSD test (α= 0.001,n= 12 forPst avrRps4andPst avrRpt2,n= 16 forPst). Data points were combined from three (Pst avrRps4,Pst avrRpt2) or four (Pst) independent experiments, each with four replicates. Note: significance codes are assigned based on the statistical analysis per treatment and should be read columnwise.bA heatmap of quantitative cell death assays conducted on leaves of indicated genotypes after infiltration utilising thePseudomonas fluorescens0–1 effector tester strain (hereafterPf0-1) delivering avrRps4 (OD600= 0.2). Cell death was measured by electrolyte leakage from bacteria-infiltrated leaf discs at 6, 8, 10 and 24 hpi. Data are displayed as means from four experiments, each with four replicates (n= 16). Statistical significance codes for the difference in means are based on Tukey’s HSD test (α= 0.001). In mutants marked in red, thePAD4–ADR1s cell death branch operates in TNLRRS1-RPS4immunity whenSAG101–NRG1s andICS1pathways are not functional. Note: significance codes are assigned based on the statistical analysis per timepoint and should be read columnwise. Boxplot representation of the same data is provided in Supplementary Figs. 5 and 6.cVisual cell death symptoms at 24 hpiPf0-1avrRps4infiltrating into leaf halves of indicated genotypes as inb. The ratio beneath each leaf indicates number of leaves with visible tissue collapse from all infiltrated leaves in two independent experiments. White arrows mark cell death visible as tissue collapse in a manner dependent onSAG101–NRG1s. Red arrows mark cell death in lines without functionalSAG101–NRG1s andICS1. Genotypes in red have functionalPAD4–ADR1sbut notSAG101–NRG1s.PstPseudomonas syringaepv.tomatoDC3000,Pf0-1 effector tester strain ofPseudomonas fluorescens0–1, CFU colony-forming units, EV empty vector. Level 1 golden gate and gateway expression constructs were transformed via electroporation into Rhizobium radiobacter (hereafter Agrobacterium tumefaciens or Agrobacteria ) GV3101 pMP90RK or pMP90 for transient expression in N. benthamiana and stable expression in Arabidopsis (Supplementary Table 2 ). We transformed pXCG pSAG101:SAG101-YFP and pAlligator2 pPAD4:YFP-Linker-PAD4 into Arabidopsis pad4-1 sag101-3 mutant and selected homozygous complementation lines using BASTA resistance or the GFP seed coat fluorescence markers, respectively. Pseudomonas growth and cell death assays in Arabidopsis Pseudomonas syringae pv. tomato ( Pst ) DC3000 with the empty vector pVSP61, pVSP61 avrRps4 or pVSP61 avrRpt2 were syringe-infiltrated into Arabidopsis leaves at OD 600 = 0.0005 in 10 mM MgCl 2 . Leaf discs were harvested at 0 dpi (four leaf discs as four replicates) and 3 dpi (12 leaf discs divided over four replicates). Biological replicates are experiments performed on different days with the same or different batches of plants. For cell death assays, a type III secretion system-equipped Pseudomonas fluorescens effector tester strain Pf 0-1 avrRps4 [48] was resuspended in 10 mM MgCl 2 (OD 600 = 0.2) and syringe-infiltrated into leaves. Only the type III secretion system-equipped and not the wild type Pf 0-1 strain was used in this study, and for simplicity, we refer to it as “ Pf 0-1”. Eight leaves per genotype were infiltrated for each biological replicate (experiments performed on different days with the same or different batches of plants). The conductivity of solution with the incubated leaf discs was measured at 6, 8, 10, and 24 hpi as described earlier [26] . Macroscopic cell death phenotype was recorded at 24 hpi. For cell death assays with Pst avrRpt2 , bacteria were resuspended 10 mM MgCl 2 to OD 600 = 0.02 and electrolyte leakage was measured as described for Pf 0-1 avrRps4 triggered cell death. The statistical analysis included checking normality of residuals distribution (Shapiro–Wilcoxon at α = 0.05 or visually with qq-plot) and homoscedasticity (Levene test at α = 0.05). Difference in means was assessed via Tukey’s HSD test ( α = 0.001, experiment taken as a factor in ANOVA). Roq1 signalling reconstitution assays in N. benthamiana Roq1 cell death reconstitution assays were performed with the Pf 0-1 XopQ [67] strain in N. benthamiana quadruple mutant eds1a pad4 sag101a sag101b ( Nb epss ) [26] . Agrobacteria induced for one hour in Agromix (10 mM MgCl 2 , 10 mM MES pH 5.6, 150 μM acetosyringone) were firstly syringe-infiltrated at OD 600 = 0.2 into Nb epss leaves. At 48 hpi, Pf 0-1 XopQ or Pf 0-1 (empty vector) were infiltrated at OD 600 = 0.3 in the same leaf zone. At 24 h after Pf 0-1 XopQ infiltration, macroscopic cell death phenotype was recorded and four-leaf discs (as four replicates) were taken for measuring electrolyte leakage at 6 h after collecting the leaf discs. Xanthomonas campestris pv. vesicatoria ( Xcv 85-10; also named Xanthomonas euvesicatoria ) growth assays in Nb epss in the presence of Agrobacteria to express proteins of interest were performed as described earlier [26] . Co-IP and immunoblotting analyses In Co-IP assays with proteins expressed in N. benthamiana Roq1 reconstitution assays, five 10 mm leaf discs were collected to form a sample. Total protein from the plant material ground to fine powder was extracted in 2 ml of the extraction buffer (10% glycerol, 100 mM Tris–HCl pH 7.5, 5 mM MgCl 2 , 300 mM NaCl, 10 mM DTT, 0.5% NP-40, 2% PVPP, 1x Plant protease cocktail (11873580001, MilliporeSigma)). Lysates were centrifuged for 35 min at 4500 × g and filtered through two layers of Miracloth (475855, MilliporeSigma). The 50 µl aliquots of the filtered supernatant were taken as input samples. Co-IP were conducted for 2 h with 12 μl α-HA affinity matrix (11815016001, MilliporeSigma) under constant rotation. Beads were collected by centrifugation at 4000 × g for 1 min and washed four times in extraction buffer (without DTT and PVPP). All co-IP steps were conducted at 4 °C. Beads and input samples were boiled at 95 °C in 100 μl 2 × Laemmli buffer for 10 min. Antibodies used for immunoblotting were α-GFP (11814460001, MilliporeSigma), α-HA (1:5000; c29f4, Cell Signalling), α-FLAG (1:5000; f1804, MilliporeSigma), HRP-conjugated antibodies (A9044 and A6154, Sigma-Aldrich; sc-2006 and sc-2005, Santa Cruz). Antibodies were used in dilution 1:5000 (TBST with 3% non-fat milk powder). Images of blots are provided in the Source data file accompanying this paper. Immunoprecipitation of EDS1-YFP and TRB1-GFP in Arabidopsis Nuclei-enriched fractions were isolated from ~20 g of leaves of 4–5 week-old plants grown under short day conditions described above and vacuum-infiltrated with Pst avrRps4 (OD 600 = 0.1, 10 mM MgCl 2 supplemented with 0.005% Silwet-L77). Samples were collected at 8–10 h after the infiltration. After sample collection, all steps were conducted at 4 °C or on ice. Extraction was performed mainly as in ref. [68] with modifications. Leaves were chopped with a razor blade, all buffers contained a 2xPlant Protease inhibitor cocktail (11873580001, MilliporeSigma). Separation was performed only on one Percoll gradient (80–30%) followed by a final clean-up through the 30% Percoll layer. Nuclei-enriched fractions were spun down for 10 min at 1000 × g to remove Percoll and hexylene glycol. The nuclei-enriched fraction was gently resuspended in 1 ml of the sample buffer (20 mM Tris–HCl pH 7.4, 2 mM MgCl 2 , 150 mM NaCl, 5% glycerol, 5 mM DTT, EDTA-free protease inhibitor (11873580001, MilliporeSigma)), centrifuged for 10 min at 1000 × g , and carefully resuspended again in 600 μl of the sample buffer. After incubation of washed nuclei at 37 °C with 10 units of DNase I (89836, Thermo Fisher Scientific) and 20 μg of RNase A (EN0531, Thermo Fisher Scientific) under soft agitation for 15 min, samples were placed on ice for 10 min and sonicated for six cycles 15 s “on”–15 s “off” using Bioruptor Plus (Diagenode). After that, samples were centrifuged for 15 min at 16,000 × g , and the supernatant was used as input for IP with GFP-trap A beads (per IP, 25 μl of slurry prewashed in 2 ml of the samples buffer, gta-100 (Proteintech)). Before IP, 25 μl of the supernatant is set aside as an input fraction for quality controls. Then, samples were supplemented with 10% Triton X-100 to the final concentration 0.1% and 0.5 M EDTA to the final concentration of 2 mM. After 2.5 h of incubation with the sample in Protein Lobind tubes (0030108116 and 0030108132, Eppendorf), beads were washed four times in 300 μl 3 min each in the wash buffer (20 mM Tris–HCl pH 7.4, 150 mM NaCl, 2 mM EDTA). Proteins were eluted in 2 × 35 μl 0.1% TFA and neutralised in 90 μl of Tris–Urea (4 M urea 50 mM Tris–HCl pH 8.5). Gel filtration chromatography Nuclear extracts (600 μl) from the pEDS1:EDS1-YFP complementation line were processed as for IP input in the subsection “Immunoprecipitation (IP) of EDS1-YFP and TRB1-GFP from respective Arabidopsis complementation lines”. Obtained samples were fractionated on the column Superose 6 10/300 GL (50 kDa–5 MDa range, GE Healthcare Life Sciences, Ӓkta FPLC) at the rate 0.5 ml/min in 20 mM Tris–HCl pH 7.4 and 150 mM NaCl. The temperature was kept at 4 °C. In total, 28 0.5 ml fractions per sample were collected, concentrated with StrataClean resin (400714, Agilent) and analysed using Western blot method (α-GFP, 11814460001, MilliporeSigma) with the same total EDS1-YFP sample on each blot for the between-blot normalisation. A high-molecular weight marker was run prior to each experiment (28403842, GE Healthcare Life Sciences). Immunoprecipitation of YFP-PAD4 and SAG101-YFP in Arabidopsis Five-week-old Arabidopsis plants containing p35S:StrepII-3xHA-YFP (Col-0), pPAD4:YFP-PAD4 ( pad4-1 sag101-3 background) or pSAG101:SAG101-YFP ( pad4-1 sag101-3 ) were vacuum infiltrated with Pf 0-1 avrRps4 bacteria (OD = 0.2 in 10 mM MgCl 2 with 0.01% Silwet L-70). ~2 g of rosette material was collected at 6 hpi, snap-frozen in liquid nitrogen and kept at −80 °C until IP. On the day of IP, samples were ground to fine powder in Precellys 15 ml tubes (P000946-LYSK0-A, Bertin Instruments). The protein extraction was performed in 10 ml of the buffer composed of 20 mM PIPES–KOH pH 7.0, 150 mM NaCl, 10 mM MgCl 2 , 10% glycerol (v/v), 5 mM DTT, 1% Triton X-100, Plant Protease Inhibitor cocktail (11873580001, MilliporeSigma). The protein extraction was performed at 4 °C for 20 min under constant end-to-end mixing (~60 rpm). After that, the samples were cleared by centrifuging 20 min at 4 °C 3000 × g . The supernatant was passed once through 0.2 μm filters (KC64.1, Roth) to remove debris. Each sample (10 ml in 15 ml Falcon tubes) was incubated for 2.5 h at 4 °C under constant end-to-end mixing (~20 rpm) with equilibrated beads corresponding to 20 μl of GFP-trapA (gta100, Proteintech) slurry. After the incubation, beads were washed three times 5 min each with the wash buffer containing 20 mM Tris–HCl pH 7.4, 150 mM NaCl, 0.01% Triton X-100, Plant Protease Inhibitor cocktail (11873580001, MilliporeSigma). Finally, to remove Triton X-100 traces, the beads were washed two additional times 1 min each in the buffer with 20 mM Tris–HCl pH 7.4 and 150 mM NaCl. Purification of NRG1.2 from the Arabidopsis complementation line Arabidopsis Ws-2 nrg1a nrg1b complementation line from [19] was grown in short-day conditions for 5–6 weeks. Pf 0-1 empty vector or Pf 0-1 avrRps4 were resuspended in the infiltration buffer (10 mM MES pH 5.7, 10 mM MgCl 2 ) at OD 600 = 0.3 and syringe-infiltrated into apoplastic space of rosette leaves. Approximately 2.5 g of tissue was harvested 4 hpi and flash frozen. Tissue was ground in liquid nitrogen before lysis in 100 mM HEPES (pH 7.5), 300 mM NaCl, 5 mM MgCl 2 , 0.5% Nonidet P-40, 10 mM DTT, 10% glycerol, and cOmplete ™ EDTA-free Protease Inhibitor Cocktail (11873580001, MilliporeSigma). Lysate was centrifuged at 4000 × g for 35 min at 4 °C and filtered through Miracloth to pellet and remove debris. Lysate was incubated with buffer equilibrated ANTI-FLAG ® M2 Affinity Agarose beads (A2220, MilliporeSigma) for 45 min. Beads were washed before incubation with 3XFLAG ® Peptide (F4799, Sigma-Aldrich) for 2 h. Eluate was collected for further analysis by immunoblot and mass spectroscopy. Immunoblot analysis of NRG1.2-EDS1 interactions in Arabidopsis Samples were heated in 4× SDS sample loading buffer (10 mM DTT) at 65 °C for 5 min. Proteins were resolved on 4–20% SDS–PAGE (4561095, Bio-Rad) and dry transferred by Trans-Blot Turbo Transfer System to PVDF membrane (170427, Bio-Rad). Membranes were blocked in 5% milk (v/w) in TBST for 1 h. For protein detection, HRP-conjugated anti-FLAG (A-8592, Sigma-Aldrich) was used at 1:30,000 (TBST, 5% milk powder [v/w]) and anti-EDS1 (AS13 2751, Agrisera) was used at 1:3000 (TBST, 3% milk powder [v/w]) and probed overnight at 4 °C. Membranes were washed three times in TBS-T for 10 min. Secondary HRP-conjugated antibody (A0545, MilliporeSigma) was used at 1:10,000 (TBST, 5% milk powder [v/w]) at RT for 2 h. Membranes were washed three times in TBST for 10 min, and three times in TBS for 5 min. 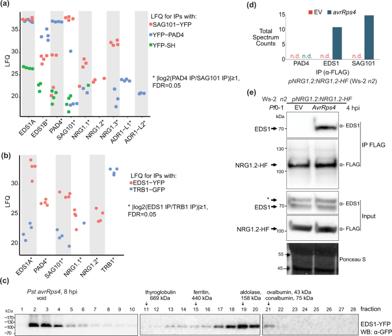Fig. 3: Early effector-dependent NRG1 association with EDS1 and SAG101 inArabidopsisTNLRRS1–RPS4triggered ETI. aDotplot of normalised abundance values (label-free quantification (LFQ), log2-scaled) for proteins detected in liquid chromatography–mass spectrometry (LC–MS) analyses after α-GFP immunoprecipitation (IP) of PAD4-YFP or SAG101-YFP from total leaf extracts of respective complementation linespPAD4:YFP-PAD4andpSAG101:SAG101-YFP(both Colpad4 sag101background) after infiltration with effector tester stra5in ofPseudomonas fluorescens0-1 (Pf0-1)avrRps4(6 hpi, OD600= 0.2). ADR1s are specifically enriched in PAD4-YFP IP samples, whereas NRG1s are more abundant in the SAG101-YFP IP samples. Samples were collected from four independent experiments.bDotplot of LFQ values for proteins detected in LC–MS analyses after IP of EDS1-YFP and TRB1-GFP from nuclei-enriched extracts of correspondingArabidopsiscomplementation lines infiltrated withPseudomonas syringaepv.tomatoDC3000 (Pst)avrRps4(8 hpi, OD600= 0.1). NRG1.1 and NRG1.2 are specifically enriched in EDS1-YFP samples. Samples were collected from four independent experiments.cα-GFP probed immunoblots of nuclei-enriched extracts from leaves of theArabidopsis pEDS1:EDS1-YFPcomplementation line (Coleds1-2background) infiltrated withPst avrRps4(OD600= 0.1, 8 hpi). Extracts were resolved using native gel filtration. Arrows below protein markers indicate position of the corresponding peak. Numbers refer to column fractions. EDS1 forms stable ~100–600 kDa complexes. The experiment was conducted three times with similar results.dLC–MS analysis of eluates after α-FLAG IP of total leaf extracts fromArabidopsisWs-2n2 pNRG1.2:NRG1.2-HFcomplementation line infiltrated withPf0-1 empty vector (EV) orPf0-1avrRps4(4 hpi, OD600= 0.3). Peptides corresponding to EDS1 and SAG101 were observed in eluates only afterPf0-1-mediated delivery of avrRps4. This result was observed in two independent experiments.eWestern blot (WB) analysis of eluates from (d). Asterisk indicates a nonspecific band on the α-EDS1 blot for input samples. The analysis was performed on total leaf extracts and was conducted four times with similar results. Association of EDS1 with NRG1.2-HF was observed only afterPf0-1-mediated delivery of avrRps4. Ponceau S staining shows similar protein loading in input samples on the blot. Detection of signal was performed with enhanced chemiluminescent horseradish peroxidase substrates SuperSignal ™ West Pico PLUS (34580, Thermo Fischer Scientific) and Femto (34095, Thermo Fischer Scientific), and ImageQuant LAS 4000 ™ for protein band visualisation. Images of blots are provided in the Source data file accompanying this paper. Arabidopsis NRG1.1 structure homology modelling NRG1.1 (AT5G66900.1) was modelled on ZAR1 resistosome cryo-electron microscopy structure (PDB: 6j5t) using SWISS-MODEL [69] (SMTL version 2019-05-22, PDB release 2019-05-17; ProMod3 v. 1.3.0). Visualisation was performed in Pymol (v. 2.3.4–2.4.1, Schrödinger, LLC). Software used for visualisation and statistical analysis of data Statistical analysis was performed in R (3.6.1 through 4.0.2) using base ANOVA and posthoc tests. Heatmaps were generated with the pheatmap (1.0.12) package in R. Boxplots and barplots were generated with the ggplot2 (3.3.2) package in R. Multiple sequence alignment in Supplementary Fig. 11 was prepared with msa package (1.22.0) in R. An NRG1.1 structure model was prepared with SWISS-MODEL [69] (SMTL version 2019-05-22, PDB release 2019-05-17; ProMod3 v. 1.3.0). Visualisation of the structures was performed in Pymol (2.3.4-2.4.1, Schrödinger, LLC). Excel in Microsoft Office suites 2016, 2019, 365 were used for the analysis of processed mass spectrometry data. 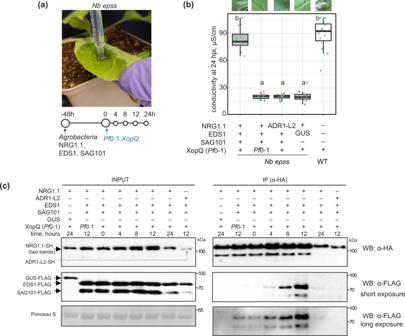Fig. 4: XopQ/Roq1-dependentArabidopsisNRG1.1 association with EDS1 and SAG101 inNicotiana benthamiana. aSample collection scheme for experiments in (b) and (c). Roq1-dependent cell death is restored inNicotiana benthamiana(Nb)eds1 pad4 sag101a sag101b(Nb epss) signalling deficient mutant by expressingArabidopsisEDS1, SAG101 and NRG1.1 viaAgrobacteriainfiltration 48 h before XopQ effector delivery.Pf0-1XopQis syringe-infiltrated (OD600= 0.3) to deliver the effector and to study TNL signalling events in a time-resolved manner up to 24 hpi.bMacroscopic symptoms and quantification of XopQ-triggered cell death at 24 hpi after infiltratingPf0-1XopQin leaves ofNb epssexpressingArabidopsisEDS1-FLAG, SAG101-FLAG, NRG1.1-3xHA-StrepII (NRG1.1-SH) or ADR1-L2-3xHA-StrepII (ADR1-L2-SH).Pf0-1 with empty vector (Pf0-1) served as a “no-ETI” control. Cell death was quantified in electrolyte leakage assays 6 h after harvesting leaf discs (24 hpi withPf0-1XopQ). The experiment was performed three times independently, each with four replicates (leaf discs) (Tukey’s HSD,α= 0.001,n= 12). Transiently expressedArabidopsisEDS1, SAG101 and NRG1.1 proteins are functional inPf0-1XopQtriggered (Roq1) cell death. Description of boxplots: minima—first quartile, maxima—third quartile, centre—median, whiskers extend to the minimum and maximum values but not further than 1.5 interquartile range from the respective minima or maxima of the boxplot. Datapoints with the same colour come from one independent experiment.cCoimmunoprecipitation assay followed by Western blotting to test for XopQ-triggered associations betweenArabidopsisNRG1.1-SH and FLAG-tagged EDS1 or SAG101 inNb epssaccording to the infiltration scheme in (a). NRG1.1-SH or ADR1-SH were enriched using α-HA agarose beads, and presence of FLAG-tagged EDS1, SAG101 or GUS was tested by probing blots with α-FLAG antibodies. IP assays were conducted three times independently with similar results. NRG1.1 association with EDS1 and SAG101 requires Roq1/XopQ ETI activation.Pf0-1 effector tester strain ofPseudomonas fluorescens0–1 with empty vector,Pf0-1XopQ(ina) or XopQ (Pf0-1) effector tester strain ofPseudomonas fluorescens0–1 deliveringXopQ, WB Western blotting, IP immunoprecipitation,Nb epssNicotiana benthamiana eds1a pad4 sag101a sag101b. 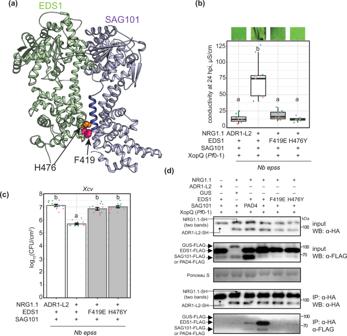Fig. 5: Effector-dependent NRG1–EDS1–SAG101 association requires a functional EDS1 EP domain. aTheArabidopsisEDS1 (green)—SAG101 (purple) heterodimer crystal structure (PDB: 4NFU) with highlighted EP domain cavity essential for TNL-triggered cell death. An α-helix of the SAG101 EP domain (blue) and residues F419 (magenta) and H476 (orange) in EDS1 EP domain are shown as ribbon and spheres, respectively.b,cRoq1/XopQ-dependent cell death (b) and bacterialXcvresistance (c) in leaves ofNb epsstransiently expressing of C-terminally FLAG-tagged EDS1 wildtype and mutant variants with SAG101-FLAG and NRG1.1-SH or ADR1-L2-SH. Cell death was triggered by infiltratingPf0-1XopQat 48 h afterAgrobacteriainfiltration; photos of leaves were taken at 24 h. F419E and H476Y mutations in theArabidopsisEDS1 EP domain abrogated cell death and resistance. Experiments were performed three times independently, each with four replicates (leaf discs) (Tukey’s HSD,α= 0.001,n= 12). Error bars represent standard error of mean. Description of boxplots: minima—first quartile, maxima—third quartile, centre—median, whiskers extend to the minimum and maximum values but not further than 1.5 inter-quartile range from respective minima or maxima of the boxplot. Datapoints with the same colour come from one independent experiment.dIP followed by Western blot analysis to test the dependency of associations betweenArabidopsisEDS1, SAG101 and NRG1.1 inNb epsson a functional EDS1 EP domain cavity. Leaves ofNb epsswere infiltrated withAgrobacteriato express FLAG-tagged EDS1 or its variants EDS1F419Eand EDS1H476Y, SAG101-FLAG and NRG1.1-SH or PAD4-FLAG, with ADR1-L2-SH and GUS-FLAG as negative controls. At 2 dpi,Pf0-1XopQ(OD600= 0.3) was infiltrated, and the triggered samples were collected at 10 hpi. Following IP with α-HA agarose beads, input and IP fractions were probed with α-HA and α-FLAG antibodies. Roq1/XopQ-dependent association of NRG1.1-SH with EDS1-FLAG and SAG101-FLAG was abolished in samples with mutated EDS1 EP domain variants. Similar results were obtained in three independent experiments.XcvXanthomonas campestrispv.vesicatoriastrain 85-10, XopQ (Pf0-1) effector tester strain ofPseudomonas fluorescens0–1 delivering XopQ, WB Western blotting, IP immunoprecipitation,Nb epssNicotiana benthamiana eds1a pad4 sag101a sag101b. 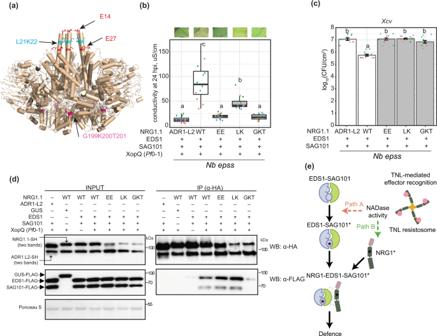Fig. 6: Association betweenArabidopsisNRG1.1, EDS1 and SAG101 require an intact NRG1.1 P-loop. aA structure homology model ofArabidopsisNRG1.1 based on the ZAR1 resistosome. NRG1.1 amino acids E14 and E27 (red sticks) and L21 and K22 (blue sticks) aligned with residues E11, E18, F9, L10 and L14 in ZAR1. The modelled NRG1.1 P-loop motif (G199 K200 T201) is shown as cyan sticks. XopQ-triggered cell death (b) andXanthomonas campestrispv.vesicatoriastrain 85-10 (Xcv) growth restriction (c) inNicotiana benthamiana eds1a pad4 sag101a sag101b(Nb epss) expressingArabidopsisNRG1.1-SH wildtype, NRG1.1E14A/E27A, NRG1.1L21A/K22Aand NRG1.1G199A/K200A/T201Avariants together with EDS1-FLAG and SAG101-FLAG.Arabidopsisproteins were expressed viaAgrobacteria-mediated transient expression assays two days before infiltration ofPseudomonas fluorescens0-1 (Pf0-1)XopQ(OD600= 0.3) or simultaneously withXcv(OD600= 0.0005). Experiments were performed three times independently, each with four replicates (leaf discs) (Tukey’s HSD,α= 0.001,n= 12). Error bars represent standard error of mean. Datapoints with the same colour come from one independent experiment.dImmunoprecipitation (IP) and Western blot (WB) analyses testing associations ofArabidopsisNRG1.1 mutant variants with EDS1 and SAG101 inNb epssafter triggering Roq1 signalling byPf0-1XopQinfiltration (OD600= 0.3; 10 hpi).ArabidopsisEDS1-FLAG, SAG101-FLAG with NRG1.1-SH, and using GUS-FLAG andArabidopsisADR1-L2-SH as negative controls, were expressed usingAgrobacteria2 d prior toPf0-1XopQinfiltration. After α-HA IP, the indicated fractions were analysed with α-HA and α-FLAG antibodies by WB. The experiment was conducted three times independently with similar results.eModel of molecular events leading to generation of anArabidopsisEDS1–SAG101–NRG1 signalling complex essential for TNL receptor-activated defence. NRG1–EDS1–SAG101 association is dependent on TNL activation and requires an intact EDS1–SAG101 heterodimer EP domain cavity (purple circle) and NRG1 nucleotide-binding domain. In two depicted scenarios, an effector-induced TNL oligomer with NADase activity leads to activation (asterisks) of EDS1–SAG101 via the EP domain cavity (‘Path A’, asterisk inside the purple circle) or NRG1 (‘Path B’). These paths are not mutually exclusive. EDS1–SAG101–NRG1 assembly precedes and is necessary for TNL-triggered cell death and resistance involving a predicted NRG1 N-terminal HeLo domain α-helix. Reporting summary Further information on research design is available in the Nature Research Reporting Summary linked to this article.